Phase evolution in single-crystalline LiFePO4followed byin situscanning X-ray microscopy of a micrometre-sized battery LiFePO 4 is one of the most frequently studied positive electrode materials for lithium-ion batteries during the last years. Nevertheless, there is still an extensive debate on the mechanism of phase transformation. On the one hand this is due to the small energetic differences involved and hence the great sensitivity with respect to parameters such as size and morphology. On the other hand this is due to the lack of in situ observations with appreciable space and time resolution. Here we present scanning transmission X-ray microscopy measurements following in situ the phase boundary propagation within a LiFePO 4 single crystal along the (010) orientation during electrochemical lithiation/delithiation. We follow, on a battery-relevant timescale, the evolution of a two-phase-front on a micrometre scale with a lateral resolution of 30 nm and with minutes of time resolution. The growth pattern is found to be dominated by elastic effects rather than being transport-controlled. LiFePO 4 (LFP) has been intensively studied for the application in Li-ion batteries because of its excellent electrode performance, low cost and environmental benignity. Despite huge efforts in analysing the phase transformation in LFP [1] , [2] , [3] , [4] , [5] , [6] , [7] , the mechanism is still not fully understood and appears to depend on various parameters, such as particle size and morphology [8] , [9] . The phase diagram for the macroscopic phases of particles larger than 100 nm indicates solubility for LFP and FePO 4 (FP) of below 10% at room temperature [9] , [10] , [11] , [12] , [13] . In between a two-phase system is energetically favourable, yet with only small excess energies (of ~50 mV (ref. 7 )) of the solid solution. Therefore, most of the proposed models for the (de)lithiation mechanism of (Li)FePO 4 involve the co-existence of two intraparticle phases [1] , [2] , [3] , [4] , [5] , [6] , although also lines of evidence for a single-phase mechanism along a solid solution pathway have been given [7] , [9] , and even presence of a staging phase has been demonstrated [14] . The reason for the various possibilities and scenarios referred to below is the small excess energy that can be easily washed out by other effects such as capillary pressure or elastic effects. In small particles the formation of an interface may already cost so much energy, that small enough nanocrystals are stable in the solid solution form. Indeed, a shrinking and eventually disappearing gap has been reported in the literature on size decrease [9] . The non-monotonic form of the chemical potential of Li leads to the fact that even in the single-phase mode potentiostatically intermediate compositions are quickly passed through. For an ensemble of many particles generally a digital phase distribution [3] can be realized without internal phase boundary. Indeed, a situation where particles are either almost completely lithiated or almost completely Li-free (corresponding to the solubility limits) has been observed [15] . For a sufficiently large single particle clearly the formation of an interface is favoured. Shrinking core but also the inverse scenario (size-dependent), as well as delithiation from only one side of the particle have been detected [2] , [16] . Chen et al. [1] identified stripe patterns with a period typical for spinodal decomposition or decomposition heavily influenced by elastic effects. Such a spinodal-like decomposition of LFP is also reported elsewhere in literature [17] and was related to a surface-reaction-limited model [18] . For very large crystal fragmentation, and loss of single crystallinity have been found [19] . The situation is additionally puzzled by the possibility of observing amorphization [20] as well as Li ordering. Aberration-corrected TEM gave evidence for Li staging at an overall occupancy of 50% (every second Li layer Li-free or fully occupied) [14] . It is noteworthy that this phenomenon corresponds to the above heterogenization on the multiparticle level; however, now on the level of individual layers in a single-particle situation. The stabilization via ordering may lead to the appearance of this Li 0.5 FePO 4 phase or ordered phases of different compositions (for example, integer multiplies of 1/6 (ref. 14 )) as kinetic or thermodynamic attractors; indeed, a metastable crystal phase Li x FePO 4 with x =0.6–0.75 was detected in ref. 21 via time-resolved XRD during (dis)charging, fitting to the eutectoid point at x =0.6 at 200 °C reported in ref. 22 using chemical delithiation. In addition, such an ordered intermediate phase may form a low-energy solution for the LFP/FP interface itself [23] . Ordering of different distinguished compositions is presented and has been indicated by modelling [23] , [24] . The situation is, furthermore, complicated by the fact, that in literature results obtained by chemical delithiation [1] , [2] , [19] , [22] and electrochemical delithiation [2] , [3] , [4] , [5] are mingled with each other, although they are not necessarily expected to provide the same results even for particles of same size and morphology, due to different heights of driving forces for the delithiation [22] , as well as due to different mechanisms of combined Li + and e − insertion. While the LFP and FP phases are crystallographically very similar, from a defect chemical point of view they—for simple reasons—behave antagonistically: while intrinsically LFP is characterized by lithium vacancies as ionic carriers and p-type electronic conduction, FP is an n-type conductor exhibiting Li interstitials as ionic defects [25] , [26] , [27] , [28] . A rather comprehensive description was given in ref. 25 . Interestingly, orientation experiments showed expectedly lowered mobilities along a (100) but unexpectedly similar values for b (010) and c (001) [27] , [29] . This can be attributed to the existence of antisite defects blocking the crystallographically easy conduction along the b axis [8] , [26] , the latter having been observed for short-range motion (see, for example, ref. 29 ). Clearly, there is an urgent need for in situ observation in a battery cell configuration with a defect chemically well-characterized single-crystalline electrode, which is not so large that just irreversible phase fragmentation is observed. Scanning transmission X-ray microscopy (STXM) is one of the eligible techniques due to its favourable combination of chemical resolution, spatial resolution, field of view, low dose and connected favourable signal-to-noise ratio and measurement time, clean UHV environment and X-ray beam transmission, enabling high-resolution imaging of LFP/FP phase propagation. While in situ XRD measurements [21] , [30] refer to ensemble averages and the forte of in situ TEM measurements [31] , [32] lies in probing smaller-length scales, STXM allows to observe the single-particle delithiation/lithiation mechanism with high chemical, spatial and time resolution on a battery-relevant overall length scale comparable to a single particle in an electrode. The LFP transformation mechanism is studied during in situ (de)lithiation using an oriented LFP single crystal with a size of 16 × 1 × 0.2 μm ( c × b × a direction) as a well-defined system, where due to the chosen thin-film battery geometry the Li + and e − fluxes are in opposite directions (see Fig. 1 ). Energy-resolved STXM is used to resolve the Fe n + charge state in situ , while electrochemically delithiating the cathode material along the (010) direction. The phase evolution is followed with a lateral resolution of 30 nm, disclosing the influence of the defect chemistry, in terms of ionic and electronic conductivities, as well as elastic effects on the (de)lithiation process. 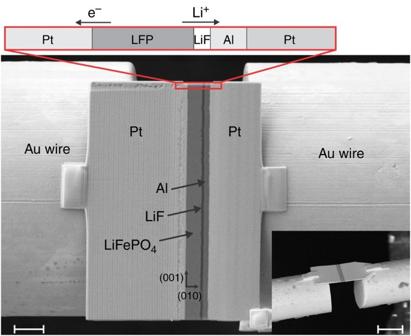Figure 1: SEM image of the micrometre-sized battery. The all-solid-state thin-film battery cell is fixed on the ends of two free-standing gold wires. During electrochemical delithiation the electron is transported to the left platinum contact, while the lithium ion is transported through the electrolyte to the aluminium anode forming a lithium–aluminium alloy there. The small inset picture shows a side view of a similar thin-film battery cell. Scale bar: 2 μm for the big SEM image, 10 μm for the small inset. Figure 1: SEM image of the micrometre-sized battery. The all-solid-state thin-film battery cell is fixed on the ends of two free-standing gold wires. During electrochemical delithiation the electron is transported to the left platinum contact, while the lithium ion is transported through the electrolyte to the aluminium anode forming a lithium–aluminium alloy there. The small inset picture shows a side view of a similar thin-film battery cell. Scale bar: 2 μm for the big SEM image, 10 μm for the small inset. Full size image Fabrication of all-solid-state micro-sized thin-film battery In order to start with most defined material conditions, LFP single crystals grown via optical floating zone technique are used [33] . Such single crystals, with dimensions on the order of millimetres, have already been carefully characterized and their defect chemistry analysed in previous publications [1] , [26] , [28] . To be able to electrochemically delithiate the material, we deposit a solid electrolyte layer (LiF) of ~100 nm on top of the previous oriented LFP single crystal using molecular beam deposition (UHV, base pressure 1 × 10 −10 mbar), followed by sputtering a 400-nm-thick layer of aluminium on top of the electrolyte as anode material. Using a focused ion beam (FIB, Ga beam) inside a scanning electron microscope (SEM, Zeiss Crossbeam) and a gaseous organoplatinum precursor we perform ion beam-induced deposition of Platinum (IBID-Pt) to deposit a platinum bar of ~3.5 μm thickness on top of this sandwich structure before cutting a 16 × 16 × 1-μm lamella sample out of this formation. In further steps we cut a cuboid cavity with dimensions 15 × 8 × 0.6 μm in the LFP part of the structure with a distance of 1 μm to the electrolyte and fill it up with IBID-Pt using four-axis micromanipulators. This provides us with a Pt-contact on the LFP side of the multilayered sample after thinning it down to 200–250 nm of thickness and removing the redundant material at the edges (some additional SEM images recorded during sample preparation are shown in Supplementary Fig. 1 ). The obtained micrometre-sized all-solid-state thin-film battery cell is then placed between the ends of two free-standing 17-μm-thick gold wires. The distance of several micrometres between the fixing points and the cathode|electrolyte|anode material ensures that no Pt is deposited on the active battery part while fixing the sample, maintaining a clean surface (see Fig. 1 ). Here it should be mentioned that, despite a thorough sample preparation electronic pathways by Pt contamination could not be completely avoided, thus reducing the open circuit voltage (OCV) to values on the order of 100 mV and giving rise to non-Faradaic by-pass currents during electrochemical cycling. Nevertheless, the additional current flow can neither influence the observed (de)lithiation mechanism, nor can it heat the sample above room temperature (additional Joule heating was estimated to be in the mK range). In addition, the mechanistic conclusions drawn below are not affected. By this geometry, we are able to analyse the (de)lithiation mechanism along the (010) direction. The thickness of the sample is chosen to secure the stability of the structure and to provide a high transparency for X-rays in the 700-eV range using for the in situ characterization the MPI-IS UHV-STXM endstation ‘MAXYMUS’ at the UE46-PGM2 undulator beamline at the Helmholtz–Zentrum Berlin for Materials and Energy/BESSY II [34] . Between preparation and characterization the sample is kept in Ar atmosphere. STXM mapping during (de)lithiation We employed STXM, measuring at a pressure of <1 × 10 −7 mbar, due to its high chemical and spatial resolution to perform in situ absorption measurements at the Fe L 3 edge. Upon delithiation of LFP a shift in the main absorption feature from ~708 to ~710 eV occurs [30] , [35] , [36] , which can be used to fingerprint the change in the local state-of-charge of the single-crystalline sample by identifying areas containing Fe 2+ and Fe 3+ , respectively. The charge and discharge of the sample is carried out potentiostatically, changing the applied voltage stepwise. The exact time–voltage profile is shown in Supplementary Fig. 2 in the Supplementary Information . It is also shown there in Supplementary Fig. 3 that the response to the steps corresponds to a quasi-stationary morphology. Recording a detailed transient response on a given voltage step appears to be out of time resolution. To visualize the delithiation kinetics, we performed area scans at single energies (704, 708.7 and 710.6 eV) while applying constant voltages. Comparing the optical densities at each point of the sample at 708.7 eV (Fe 2+ ) and 710.6 eV (Fe 3+ ; centroids of the respective Fe 2+ and Fe 3+ Gaussian XANES contributions as previously determined by a full absorption spectrum; 704 eV used for normalization) with each other according to as a function of time and increasing voltage, records the transition between the two oxidation states and therefore the (de)lithiation of LFP. Practically, the time needed to acquire one set of images is ~8 min. A short video sequence containing all 37 images of related optical densities taken during (de)lithiation of the battery cell shows the whole delithiation/lithiation process (see Supplementary Movie 1 ). Six out of these thirty-seven images are chosen to analyse the observations in more detail and are shown in Fig. 2b,c , while line scan analysis has been performed on another 12 images providing more detailed information on the mechanism and morphology of the growth structure (see Fig. 3 ). 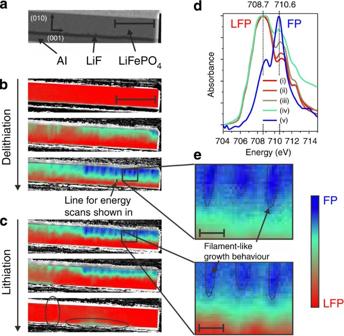Figure 2: STXM images showing the filament-like growth behaviour. (a) SEM image of the analysed region before performing STXM measurements. (b,c) STXM images comparing the optical densities of the sample at 708.7 and 710.6 eV with each other during electrochemical delithiation (b) and lithiation (c). The region of interest is colour-coded going from red (LiFePO4) over green to blue (FePO4). In the lowest image incthe begin of a crack formation along the (001) plane as well as the reversal of the Li concentration gradient upon lithiation are encircled. (d) Energy spectra taken across the borderline of the phase front along the (010) direction with (i) being recorded in the still pure LiFePO4zone, while (ii–iv) are recorded in intervals of 80 nm across the phase front (indicated in the lowest image inb) and (v) showing an energy spectrum of a fully delithiated sample with the expected absorption features of FePO4. The colour-coding of the energy spectra are carried out according to the STXM images (b,c). (e) Enlarged region of two STXM images to point out the filament-like growth behaviour of FP in LFP (upper image) and the rather homogeneous receding of FP in LFP (lower image). Scale bar: 2 μm ina,b, 200 nm ine. Figure 2: STXM images showing the filament-like growth behaviour. ( a ) SEM image of the analysed region before performing STXM measurements. ( b , c ) STXM images comparing the optical densities of the sample at 708.7 and 710.6 eV with each other during electrochemical delithiation ( b ) and lithiation ( c ). The region of interest is colour-coded going from red (LiFePO 4 ) over green to blue (FePO 4 ). In the lowest image in c the begin of a crack formation along the (001) plane as well as the reversal of the Li concentration gradient upon lithiation are encircled. ( d ) Energy spectra taken across the borderline of the phase front along the (010) direction with (i) being recorded in the still pure LiFePO 4 zone, while (ii–iv) are recorded in intervals of 80 nm across the phase front (indicated in the lowest image in b ) and (v) showing an energy spectrum of a fully delithiated sample with the expected absorption features of FePO 4 . The colour-coding of the energy spectra are carried out according to the STXM images ( b,c ). ( e ) Enlarged region of two STXM images to point out the filament-like growth behaviour of FP in LFP (upper image) and the rather homogeneous receding of FP in LFP (lower image). Scale bar: 2 μm in a , b , 200 nm in e . 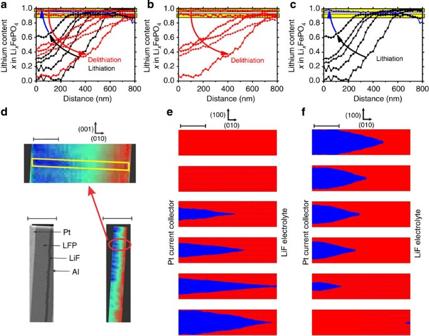Figure 3: Growth morphology of a filament. (a–c) Line scans taken at the evolving filament shown ind, giving the lithium content of the sample along the filament during delithiation (red lines ina,b) and lithiation (black lines ina,c), as well as the blue line showing the final state of the sample, including the reversal of the Li concentration gradient. (e,f) Show cross-sections of the sample at a given position of the (001) direction where the line scans have been performed (seed)). For simplicity, a symmetric filament evolution along the (100) direction is assumed during delithiation (e) and lithiation (f). Red areas indicate LFP, blue areas FP and the blue dots in the red areas dissolved FP. Scale bar: 2 μm for the lower two scale bars indand 200 nm for the upper scale bar indas well as for the scale bars ine,f. Full size image Figure 3: Growth morphology of a filament. ( a – c ) Line scans taken at the evolving filament shown in d , giving the lithium content of the sample along the filament during delithiation (red lines in a , b ) and lithiation (black lines in a , c ), as well as the blue line showing the final state of the sample, including the reversal of the Li concentration gradient. ( e , f ) Show cross-sections of the sample at a given position of the (001) direction where the line scans have been performed (see d )). For simplicity, a symmetric filament evolution along the (100) direction is assumed during delithiation ( e ) and lithiation ( f ). Red areas indicate LFP, blue areas FP and the blue dots in the red areas dissolved FP. Scale bar: 2 μm for the lower two scale bars in d and 200 nm for the upper scale bar in d as well as for the scale bars in e , f . Full size image Energy spectra recorded across the phase front at a fixed voltage illustrate the transition from LFP to Li 1− x FePO 4 /FePO 4 along the (010) direction, shown in Fig. 2d . The spectra were taken in intervals of 80 nm along the line showing a constant increase in Fe 3+ concentration. Furthermore, the energy spectra allow us to assign to the colour-coded regions in Fig. 2 , as well as to the line scans in Fig. 3 , the corresponding averaged lithium concentrations. In the images shown in Fig. 2b,c,e the red region is pure LFP, while the emerging green and blue areas indicate delithiated material. Two main characteristics during (de)lithiation are observed. First, upon delithiating the electrode material, the growing FP phase forms at the current collector side rather than at the LFP/LiF interface, while lithiation of the delithiated cathode material leads again to a growing LFP region at the electrolyte side under a retracting movement of the delithiated phase. Second, it can be seen that the delithiation of the LFP cathode material of the microbattery cell does not occur homogeneously over the whole length of the sample, resulting in a flat two-phase boundary, but rather multiple filaments of delithiated material develop along c and grow along b and a . Growth morphology of the evolving electroactive phases Before we discuss these observations in the light of ionic and electronic transport as well as elastic effects, let us have a closer look on the growth morphology of such an evolving filament as a function of time and applied voltage steps, respectively. To do so we analyse line scans taken along an evolving filament in the STXM images, shown in Fig. 3a–c ), giving the lithium content of the sample along this filament during (de)lithiation. As the sample dimension in the a direction is similar to the typical filament width, we assume single filaments in this direction as the most probable situation (cf. Fig. 3e,f ). The whole lithiation/delithiation process can be subdivided into a few main steps. In the first step, the lithium concentration is lowered over the whole length of the sample to ~90% (lower yellow marked region in Fig. 3a–c ), which is well in line with the solubility limit of FP in LFP of up to 10% at room temperature [9] , [10] , [11] , [12] , [13] . Going further up in voltage, the growth of the FP filament starts at the current collector side and is mainly growing along the b direction until it reaches the electrolyte side. Only then a more pronounced growth in the a direction starts, which can be understood in terms of the different ionic conductivities along the a and b directions [26] , [28] , [37] . During the filament-like growth of FP, the concentration of dissolved FP in the LFP phase stays at ~10%. This growth morphology is visualized in Fig. 3e ), giving cross-sections of the sample at a given position of the (001) direction where the line scans have been performed. The absence of distinct kinks in the curves confirm the above-mentioned inhomogeneity in a direction, which in Fig. 3e,f ) is represented by the assumption of a symmetrical filament. It should be kept in mind that, although we have a lateral resolution of down to 30 nm, we average at every point along the sample thickness (200–250 nm) in the direction of the beam (that is, along a ) and have no further local information on the distribution along a . In Fig. 3e,f ), the red areas indicate LFP, blue areas FP and the blue dots in the red areas dissolved FP in LFP. After reversal of current, the lithium concentration in the LFP phase increases to nominally 1, while the FP filament starts to recede from the electrolyte side (see also Fig. 3f ). The receding of the filament is again fast along the b direction and slower along a . Before the FP filament is completely lithiated, again the LFP phase shows ~10% of dissolved FP, so that it seems that the last part of the filament is dissolved in the LFP sample. The final state (blue line in Fig. 3a,c ) shows a stoichiometry polarization because obviously not all the Li removed from LFP upon delithiation could be reversibly transferred back from the Al counterelectrode. Let us now discuss the phase formation and growth morphology in terms of ionic and electronic transport as well as elastic effects. The start of delithiation and FP phase formation at the LFP-current collector contact rather than at the LFP/LiF interface indicates faster ion than electron transport σ ion (LFP)> σ eon (LFP) along b in LFP (see Fig. 4 ). 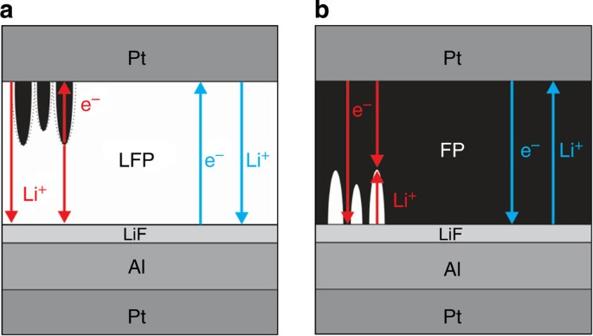Figure 4: Illustration of the phase formation requirement. This figure shows a scheme for the delithiation of LFP (a) and lithiation of FP (b). The blue arrows in the images indicate thatσeon(LFP) versusσion(LFP) (a) andσeon(FP) versusσion(FP) (b) determines on which side of the sample the (de)lithiation starts. The red arrows in both pictures clarify, that for a transport-controlled (de)lithiation one would expect homogeneous growth of FP in LFP, while filament-like growth of LFP in FP, sinceσion(LFP)>σeon(FP). Figure 4: Illustration of the phase formation requirement. This figure shows a scheme for the delithiation of LFP ( a ) and lithiation of FP ( b ). The blue arrows in the images indicate that σ eon (LFP) versus σ ion (LFP) ( a ) and σ eon (FP) versus σ ion (FP) ( b ) determines on which side of the sample the (de)lithiation starts. The red arrows in both pictures clarify, that for a transport-controlled (de)lithiation one would expect homogeneous growth of FP in LFP, while filament-like growth of LFP in FP, since σ ion (LFP)> σ eon (FP). Full size image While this is expected for an ideally intrinsic material, for the same single crystal a predominant electronic conduction was measured ( T >400 K) due to the antisite defects present, hindering ideal channel transport in realistic materials [8] , [26] , [38] . As the antisite defect concentration is not so small that the examined dimensions are below the effective distance between them, we have to seek the explanation in an enhanced donor concentration, due to the Ga beam treatment, and the lower measurement temperature (300 K). Amin et al. [39] , [40] studied the effect of a 1% Al donor-doped LFP ( (Kröger–Vink notation) act as donors) on the electronic and ionic conductivities. Their results are in agreement with the donor effect in a p-type electronic and Li-vacancy-type ionic conductor such as LFP, showing an increased ionic and a decreased electronic conductivity (compare Fig. 5 ). In addition, measuring at room temperature definitely leads to a further decrease in the hole concentration since lowering temperature favours trapping of the holes by , while the latter concentration is approximately fixed by the dopant. In fact, the trapping energy (−0.6 eV) is large enough (together with the hole-hopping energy) to compensate for the vacancy-hopping energy (for details see refs 25 , 39 , 40 , 41 ). 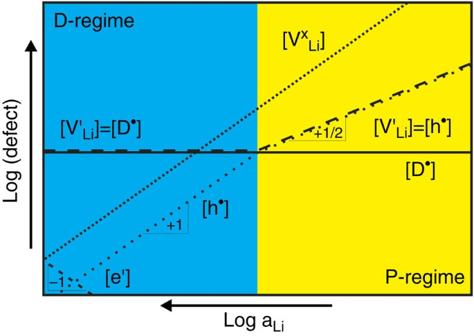Figure 5: Kröger–Vink diagram. Illustration of the defect concentration as a function of lithium activity in LFP (according to ref.25). Therefore, the faster ion than electron transport σ ion (LFP)> σ eon (LFP) along b in LFP can be understood considering the donor doping and the comparably low measuring temperature of ~300 K. Figure 5: Kröger–Vink diagram. Illustration of the defect concentration as a function of lithium activity in LFP (according to ref. 25 ). Full size image While in LFP Ga-doping enlarges Li conductivity σ ion (LFP) and decreases electronic conductivity σ eon (LFP), in the n-type electronic and Li-ion conductor FP, Ga would not be electrically active ( ) or if acting as donor ( ) further increase electronic σ eon (FP) and decrease ionic conductivity σ ion (FP). It is worth noting that such an extrinsic effect shifts defect concentrations but does not influence the quality of the defect chemical interpretation. It rather does good service in defining the defect chemical situation. Hence, the position where the delithiation of LFP and lithiation of FP starts can well be understood in terms of defect chemistry expressed in the findings that σ ion (LFP)> σ eon (LFP) and σ eon (FP)> σ ion (FP), whereat the donor concentrations do not need to be as high as the Li defiency/excess as a large fraction is realized by neutral Li defects (compare Fig. 5 ). Strikingly, upon delithiation the FP grows filament-like in the b direction. Was it the ratio of electronic to ionic conductivities in the initial phase ( σ eon (LFP)/ σ ion (LFP)) that decided upon the starting position, so is it now the ratio of ionic to electronic conductivities in the two different phases LFP and FP ( σ ion (LFP)/ σ eon (FP)) forming the criterion for growth morphology, if transport-controlled (compare Fig. 4 ). Therefore, if transport-controlled one would expect homogeneous growth of FP, as according to literature [26] , [27] and the above considerations the ionic conductivity along the b axis in LFP should exceed the electronic conductivity in FP (compare Fig. 4 ). Any thickness variation λ (thickness L ± λ ) would level out owing to the Lyapunov stability criterion if solely based on transport properties. Yet, elastic effects offer a straightforward explanation. Note that the lattice parameters for LFP with a =10.334 Å, b =6.008 Å, c =4.693 Å [42] (Pnma space group) pronouncedly differ from that of FP with a =9.821 Å, b =5.792 Å, c =4.788 Å [42] , forcing the lattice to laterally expand in the c direction. Thus, elastic effects favour an exclusion zone around the FP nuclei, which prevents further nucleation of FP phase within the vicinity and hence causes a growth pattern, which is characterized by almost regularly spaced filaments. Therefore, although small nonuniformities of the sample and therefore of the local driving force cannot totally be excluded, we can attribute this nonhomogeneous delithiation to elastic effects. It is striking that the spacing of ~200 nm is on the expected order of magnitude [1] , [43] and also observed in ref. 44 , as the distance at which mechanical failure appears upon cycling in single-crystalline LFP of comparable thickness with respect to our battery cell (extension in crystallographic a direction). This very effect can explain the filament-like growth observed very well. Owing to increased elastic strain, the filament-like growth becomes increasingly difficult and the overvoltage necessary for phase propagation exceeds well the expected value from the variation of the electrical resistance (charging to voltages up to 7 V, where a first crack along the (001) plane in the sample became visible (see Fig. 2 )). It is obvious from Figs 2b and 3b that now the filaments appear darker blue and expand in the a direction, respectively, while their length remains almost the same. Note that additional FP formation in this direction will not be stress-limited due to the comparatively thin sample (200–250 nm), which is on the order of the critical elastic thickness. The increased stress when the filaments grow along c is also reflected by the crack encircled in the lowest picture in Fig. 2c on the left side, formed upon delithiation. This is well consistent with the finding that large single crystals of LFP disintegrate on deep delithiation [20] and a performance increase upon cycling can be observed [45] . After reversal of current to prevent irreversible fragmentation (a further delithiated sample of same orientation displayed several cracks, all oriented along the (001) plane, as shown in Supplementary Fig. 4 ), again the starting points of the LFP phase growth is in line with the conductivities ( σ eon (FP)> σ ion (FP)). Moreover, again the growth morphology is opposite to what is expected from transport criteria but in line with elastic considerations. The receding of the FP is characterized by a rather homogeneous motion and not by filament-like growth of LFP expected from σ ion (LFP)> σ eon (FP) (cf. if solely based on transport properties). Obviously, again elastic effects dominate. Finally, the electrode turns completely into LFP. Only at the phase boundary to LiF now a reduction is observed due to the already mentioned incomplete transfer of the removed lithium back from the Al counter electrode leading ultimately to a reversal of the Li concentration gradient as marked in the lowest picture in Fig. 2c by the right circle. The fact that the filament structures are not homogeneous in the direction of the beam as sketched in Fig. 3e,f ) is obvious from line scans that show phase evolution at constant voltage steps. The absence of clear discontinuities can be attributed to such inhomogeneities rather than to compositional anomalies. To summarize, we succeeded in fabricating a micrometre-sized all-solid-state battery cell with oriented LFP/FP as positive electrode. We used STXM with its high chemical and spatial resolution to follow in situ the electrochemical delithiation of LFP and lithiation of FP on a micrometre scale along the fast (010) direction. The material under study is single-crystalline and its defect chemistry well understood from previous work. It is worth emphasizing that this aspect is crucial for arriving at the overall statements. The starting point of phase transformation is dictated by the respective conductivities reflecting the defect chemical situation. The growth pattern of both LFP and FP was clearly found to be dominated by elastic effects rather than being transport-controlled. This conclusion is rather general and should not depend on the exact defect chemical window. The redox reaction occurred reversibly up to a certain thickness, while more extended (galvanostatic) conditions lead to crack formation. From the filament-like pattern observed a thickness of about a few tens of nanometres seems optimal for avoiding—in a multigrain arrangement—phase separation within an individual grain and possible fracture as a result. The presented experimental approach enables an in situ recording of the phase evolution during charge–discharge of LFP/FP electrode in a battery cell. STXM proved to be very well suited for such a study owing to its high lateral and chemical resolution and may well be applied also for in situ investigations of other battery and fuel cell materials. Preparation of the micro-sized thin-film battery The LFP single crystal was grown in an optical floating zone furnace from Crystal System Incorporation at a sequential growth rate of 2 and 4 mm h −1 under a continuous argon flow, using pure phase polycrystalline LFP powder to form the feed rod (for more details see ref. 33 ). Using Laue diffraction, a slice of the single-crystalline rod was cut out exhibiting a (010) surface orientation with edges along (100) and (001). Polishing the surface with an oil–diamond suspension and cleaning it consecutively in acetone, iso-propanol and bi-distilled water in an ultrasonic bath for 15–30 min, the single crystal was transferred to the chamber for molecular beam deposition of the solid electrolyte layer (LiF). The evaporation source containing pure LiF was heated up to 820 °C to provide a beam flux of 5 × 10 −7 mbar at a base pressure of 1 × 10 −10 mbar, resulting in a growth rate of ~0.5 Å s −1 LiF on the LFP single crystal, held at room temperature. Afterwards, 400 nm aluminium was deposited via e-beam evaporation in a Univex 450 system with a base pressure of 5 × 10 −6 mbar in N 2 atmosphere. The layered structure was transferred to a Zeiss Crossbeam SEM with built-in FIB (Ga source), a positionable nozzle providing a gaseous organoplatinum precursor and a four-axis micromanipulator attached at the walls of the SEM chamber to take up the micro-sized sample and to position and align it in the electron and ion beam, respectively. A description of the sequence of the production steps is given in the section ‘Fabrication of all-solid-state micro-sized thin-film battery’ and even more detailed explanations and images of the production steps are given in Supplementary Fig. 1 . The two free-standing 17-μm-thick gold wires, between which the micrometre-sized all-solid-state thin-film battery cell was placed, were made by cutting a single gold wire with FIB. The wire was earlier positioned over a 1 × 0.2 mm wide slit in a quartz crystal, which in turn was mounted on a sample holder with two SMP-PCB adapters, connected to the gold wires, to allow for electrochemical (de)lithiation of the battery cell, while performing the STXM measurements. Between the processes of layer deposition, FIB preparation and battery characterization, the sample was kept in Ar atmosphere. STXM experiments The STXM imaging was conducted at the UE46-PGM2 undulator beamline at the Helmholtz–Zentrum Berlin for Materials and Energy/BESSY II at the so-called ‘MAXYMUS’ endstation with a provided energy range of 130–2,000 eV. We used a zone plate with a 25-nm outer zone width in whose point focus the sample, mounted on a piezo stage, was scanned by moving it perpendicular to the beam direction, while the order-sorting aperture between zone plate and sample prevents the sample from being hit from zero-order light. The total transmitted beam was detected with a fast avalanche photodetector, allowing one to extract spatial resolved spectroscopic information with a good signal-to-noise ratio as well as to perform time-resolved microscopy. All STXM measurements were performed at a pressure of <1 × 10 −7 mbar, and the charging and discharging of the all-solid-state micro-sized battery is carried out potentiostatically using a Keithley 2634B System SourceMeter. Full absorption XANES spectra were recorded between 700 and 720 eV around the Fe L 3 edge, with energy steps of 0.1 eV and a dwell time per energy step of 1,000 ms, at different positions and at different charging states of the sample to obtain reference spectra (XANES spectra of an as-prepared and a fully delithiated sample) and to assign to the differently charged regions the corresponding averaged lithium concentrations by a linear fit procedure of the normalized reference spectra. The shift in the main absorption feature from 708.7 to 710.6 eV (centroids of the respective Fe 2+ and Fe 3+ Gaussian XANES contributions) upon delithiation was used to fingerprint the change in the local state-of-charge. To visualize the phase evolution we used a field of view of 7 × 2 μm 2 scanning the sample unidirectionally at energies of 704, 708.7 and 710.6 eV with a step size of 20 nm, a dwell time at each step of 1 ms, a line delay of 250 ms and a 30-nm point focus of the X-ray beam. Comparing the optical densities at each point of the sample at 708.7 eV (Fe 2+ ) and 710.6 eV (Fe 3+ ; 704 eV used for normalization) with each other according to as a function of time and increased voltage, records the transition between the two oxidation states and therefore the (de)lithiation of LFP. The results and conclusions, based on the (de)lithiation of several micro-sized batteries of same orientation, are well reproducible. How to cite this article : Ohmer, N. et al. Phase evolution in single-crystalline LiFePO 4 followed by in situ scanning X-ray microscopy of a micrometre-sized battery. Nat. Commun. 6:6045 doi: 10.1038/ncomms7045 (2015).